A squalene synthase-like enzyme initiates production of tetraterpenoid hydrocarbons inBotryococcus brauniiRace L The green microalga Botryococcus braunii is considered a promising biofuel feedstock producer due to its prodigious accumulation of hydrocarbon oils that can be converted into fuels. B. braunii Race L produces the C 40 tetraterpenoid hydrocarbon lycopadiene via an uncharacterized biosynthetic pathway. Structural similarities suggest this pathway follows a biosynthetic mechanism analogous to that of C 30 squalene. Confirming this hypothesis, the current study identifies C 20 geranylgeranyl diphosphate (GGPP) as a precursor for lycopaoctaene biosynthesis, the first committed intermediate in the production of lycopadiene. Two squalene synthase ( SS )-like complementary DNAs are identified in race L with one encoding a true SS and the other encoding an enzyme with lycopaoctaene synthase (LOS) activity. Interestingly, LOS uses alternative C 15 and C 20 prenyl diphosphate substrates to produce combinatorial hybrid hydrocarbons, but almost exclusively uses GGPP in vivo . This discovery highlights how SS enzyme diversification results in the production of specialized tetraterpenoid oils in race L of B. braunii . Microalgae are a promising next-generation source of feedstocks for biofuel production with the potential to serve as a practical alternative to petroleum-based transportation fuels [1] . Depending on the microalgal species, the oils produced vary from triacylglycerols to hydrocarbons [2] , [3] . Hydrocarbon-based fuels are preferred over other biofuels, as they are highly compatible with existing petroleum infrastructures and possess superior fuel properties [4] , [5] . The colony-forming green microalga B. braunii is an exciting candidate for biofuel feedstock production, as it produces up to 61% of its dry weight as liquid hydrocarbon oils [6] . These hydrocarbons are produced inside the cells of the colony, seen as intracellular oil bodies and secreted into the colony extracellular matrix where the majority of the hydrocarbons are stored [6] ( Fig. 1a ). Most importantly, catalytic hydrocracking of hydrocarbons from this alga results in petroleum-equivalent fuels of gasoline, kerosene and diesel [7] . Intriguingly, geologic evidence also shows a direct contribution of this alga to the formation of currently used fossil fuel deposits around the globe [8] , [9] , [10] , [11] , [12] . Despite the aforementioned advantages of B. braunii , its use for biofuel feedstock production is hindered by a slow growth rate and the lack of transformation systems to achieve targeted genetic modification [3] . Thus, the identification of B. braunii hydrocarbon biosynthetic pathways and associated genes/enzymes can provide options for metabolically engineering these pathways into heterologous hosts with better growth characteristics and the ability to be genetically manipulated. This would then allow the development of improved versions of hydrocarbon biosynthetic enzymes, to direct production towards the most commercially desirable products [13] . 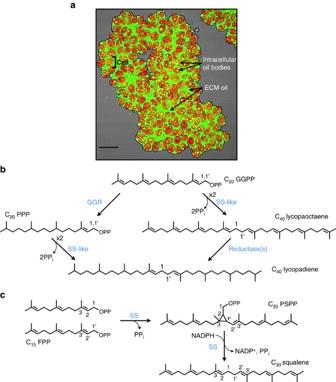Figure 1: Background information on lycopadiene biosynthesis inB. brauniirace L. (a) Confocal microscopy image of an L race colony ofB. braunii. Shown are hydrocarbon oils stained using the neutral lipid-binding stain Nile red (false coloured green) and chlorophyll autofluorescence (red). Indicated are intracellular hydrocarbon oil bodies, hydrocarbon oil in the extracellular matrix (ECM) and an individual cell as defined by chlorophyll autofluorescence from the single chloroplast in each cell. Image is an overlay of Nile red signal, chlorophyll autofluorescence signal and a bright-field image. Scale bar, 20μm. (b) Two possible pathways for lycopadiene biosynthesis. Possibility 1: GGPP reduction to PPP followed by condensation of two PPP molecules, to directly produce lycopadiene. Possibility 2: condensation of two molecules of GGPP to form lycopaoctaene, which would then be reduced to lycopadiene. (c) Two-step reaction catalysed by single SS enzyme: two molecules of FPP are condensed to squalene through the PSPP intermediate. Inbandc, enzyme names are coloured blue. Figure 1: Background information on lycopadiene biosynthesis in B. braunii race L. ( a ) Confocal microscopy image of an L race colony of B. braunii . Shown are hydrocarbon oils stained using the neutral lipid-binding stain Nile red (false coloured green) and chlorophyll autofluorescence (red). Indicated are intracellular hydrocarbon oil bodies, hydrocarbon oil in the extracellular matrix (ECM) and an individual cell as defined by chlorophyll autofluorescence from the single chloroplast in each cell. Image is an overlay of Nile red signal, chlorophyll autofluorescence signal and a bright-field image. Scale bar, 20μm. ( b ) Two possible pathways for lycopadiene biosynthesis. Possibility 1: GGPP reduction to PPP followed by condensation of two PPP molecules, to directly produce lycopadiene. Possibility 2: condensation of two molecules of GGPP to form lycopaoctaene, which would then be reduced to lycopadiene. ( c ) Two-step reaction catalysed by single SS enzyme: two molecules of FPP are condensed to squalene through the PSPP intermediate. In b and c , enzyme names are coloured blue. Full size image There are three different races of B. braunii based on the hydrocarbons synthesized. Race A produces fatty acid-derived C 23 –C 33 alkadienes and alkatrienes. Races B and L produce isoprenoid-derived hydrocarbons: methylsqualenes and C 30 –C 37 botryococcene triterpenoids in race B and the C 40 tetraterpenoid lycopadiene, the focus of this study, in race L [6] . Green algae have been shown to possess only the plastid-localized methyl erythritol phosphate pathway to supply isoprenoid precursors for terpene production [14] , [15] , and thus lycopadiene is predicted to be generated from C 5 precursors via this route. However, the exact mechanism of lycopadiene biosynthesis from C 20 prenyl diphosphate intermediates has been a mystery and two possible biosynthetic routes have been suggested ( Fig. 1b ) [16] . The first entails C 20 geranylgeranyl diphosphate (GGPP) reduction by GGPP reductase to produce C 20 phytyl diphosphate (PPP; Fig. 1b ). Two molecules of PPP would then undergo head-to-head condensation (1-1′ linkage) to produce lycopadiene ( Fig. 1b ). The second possibility is the head-to-head condensation of two GGPP molecules to produce lycopaoctaene, followed by stepwise enzymatic reduction to produce lycopadiene ( Fig. 1b ). Using either proposed route, the condensation of PPP or GGPP is predicted to proceed in a reaction mechanism similar to that carried out by the enzyme squalene synthase (SS), which forms C 30 squalene, a precursor required for sterol biosynthesis in eukaryotes [17] and hopanoids in some prokaryotes [18] . SS enzymes catalyse a two-step reaction. First, the condensation of two C 15 farnesyl diphosphate (FPP) molecules yields the cyclopropyl intermediate presqualene diphosphate (PSPP; Fig. 1c ). Second, PSPP undergoes NADPH-dependent reductive rearrangement to form squalene with a 1-1′ linkage between the two FPP molecules ( Fig. 1c ) [19] . Herein we report the elucidation of the first committed step in the lycopadiene hydrocarbon biosynthetic pathway in B. braunii Race L, which is catalysed by a new SS-like (SSL) enzyme. L race hydrocarbon content and related enzyme activity Previous studies reported trans,trans -lycopadiene as the predominant hydrocarbon (98% of total hydrocarbons) produced by race L, with a small amount of lycopatriene also documented [16] , [20] , [21] . However, the lycopatriene structure was not determined. Thus, we first set out to ascertain and refine the hydrocarbon profile of B. braunii Race L, to provide a baseline for our biosynthetic models. Analysis of purified hydrocarbons by gas chromatography–mass spectrometry (GC–MS) showed that lycopadiene accounts for 95% of the total hydrocarbon pool ( Fig. 2a (I)), with six other minor compounds constituting the remaining 5%: lycopatriene, lycopatetraene, lycopapentaene, lycopapentaene isomer, lycopahexaene and a C 35 H 64 molecule ( Fig. 2a (II–VII) and Supplementary Figs 1–4 ). Ozonolysis experiments suggested lycopatriene and lycopapentaene share an identical reduced C 20 moiety with lycopadiene ( Supplementary Figs 5–7 ). Nuclear magnetic resonance (NMR) spectroscopy was used to confirm identity and structure, including double bond positions, of each molecule ( Fig. 2a , Supplementary Table 1 and Supplementary Figs 8–15 ). This is the first report of lycopatetraene, lycopapentaene and lycopahexaene hydrocarbons from B. braunii race L. The lack of detectable amounts of lycopaoctaene and lycopaheptaene in the total hydrocarbon fraction could be due to rapid conversion of these metabolites into more highly saturated homologues. Interestingly, the unique C 35 H 64 isoprenoid hydrocarbon detected contains seven isoprene units and thus is assigned to the recently named C 35 terpene class ‘sesquarterpenes’ [22] . 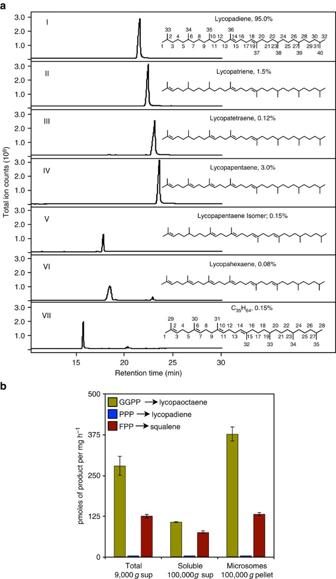Figure 2: Hydrocarbon composition and hydrocarbon-related enzyme activities inB. brauniirace L. (a) Representative GC–MS profiles of purified hydrocarbons and their corresponding names and structures (I–VII). Structures of hydrocarbons were determined by1H- and13C-NMR. Lycopadiene carbon numbering (I) is used for numbering all C40hydrocarbons of race L. Percentage next to the name of each hydrocarbon corresponds to its average amount present in total hydrocarbon pool from three independent culture cycles (n=3). (b) Radioactive enzyme assays were conducted using different protein fractions of race L cell lysates to test the two possible lycopadiene biosynthetic pathways. Enzyme activities were calculated based on the incorporation of3H-GGPP into lycopaoctaene,3H-PPP into lycopadiene and3H-FPP into squalene. SS enzyme activity is used as a positive control. Values shown are the mean±s.e. obtained from three independent experiments (n=3). Figure 2: Hydrocarbon composition and hydrocarbon-related enzyme activities in B. braunii race L. ( a ) Representative GC–MS profiles of purified hydrocarbons and their corresponding names and structures (I–VII). Structures of hydrocarbons were determined by 1 H- and 13 C-NMR. Lycopadiene carbon numbering (I) is used for numbering all C 40 hydrocarbons of race L. Percentage next to the name of each hydrocarbon corresponds to its average amount present in total hydrocarbon pool from three independent culture cycles ( n =3). ( b ) Radioactive enzyme assays were conducted using different protein fractions of race L cell lysates to test the two possible lycopadiene biosynthetic pathways. Enzyme activities were calculated based on the incorporation of 3 H-GGPP into lycopaoctaene, 3 H-PPP into lycopadiene and 3 H-FPP into squalene. SS enzyme activity is used as a positive control. Values shown are the mean±s.e. obtained from three independent experiments ( n =3). Full size image To gain more insight into the mechanism of lycopadiene biosynthesis and assess the validity of the two possible lycopadiene biosynthetic routes ( Fig. 1b ), a cell-free in vitro enzyme assay was developed using total, soluble and microsomal protein fractions with 3 H-labelled PPP and GGPP substrates for potential incorporation into lycopadiene and lycopaoctaene, respectively. Squalene production by SS enzyme activity with 3 H-labelled FPP as substrate was used as a control [23] . Lycopadiene production from PPP was not detected in any protein fraction tested, whereas lycopaoctaene biosynthesis from GGPP was easily observed, mainly in the microsomal fraction ( Fig. 2b ). This indicates a lycopaoctaene synthase (LOS) activity is localized to a membrane system, possibly the endoplasmic reticulum (ER) as is seen for SS [24] . Tellingly, LOS activity in these assays was detected when using the same cofactor and divalent metal cation as those used for SS activity measurement. These results suggest direct lycopadiene biosynthesis from PPP is not a significant contributor to C 40 hydrocarbon production in race L, whereas conversion of GGPP into lycopaoctaene occurs readily, as proposed in the second hypothetical route ( Fig. 1b ). Correspondingly, LOS enzyme activity directly correlated with lycopadiene accumulation over the growth cycle, suggesting this activity is related to hydrocarbon biosynthesis ( Supplementary Fig. 16 ). Detection of LOS activity from an algal homogenate in an assay similar to that of SS supports the notion that an LOS enzyme may be similar to a typical SS enzyme. Identification of an LOS enzyme To identify the gene(s) responsible for lycopaoctaene biosynthesis, we generated and computationally screened an L race transcriptomic database for SSL sequences. Two SSL cDNAs were identified and named based on the function of their encoded proteins as detailed below: SS from race L ( LSS ) and LOS . Both the LSS and LOS proteins contain all five conserved activity domains, the transmembrane domain and the NADPH-binding residues found in typical SS enzymes ( Supplementary Figs 17 and 18 ) [17] . Comparison of the encoded amino acid sequences showed 57.5 and 49.2% identity to SS from race B (BSS) [25] for LSS and LOS, respectively ( Supplementary Fig. 17 ). In addition, comparison of LOS with other SS and SSL enzymes showed 52.5% identity to LSS, 47.3% identity to the Solanum lycopersicum (tomato) SS ( Sl SS), 44.6, 61.7 and 44.1% identity to the SSL-1, -2 and -3 from the B race of B. braunii , and 33.9% identity to the human SS (HSS; Supplementary Fig. 18 ). Several studies [17] , [26] , [27] , [28] , including the recent determination of the crystal structure of HSS [29] , have elucidated the catalytic mechanism of the SS reaction. These studies have shown the FLAP domain, domains I–V and the JK loop of HSS form the SS active site [29] . Furthermore, several HSS residues (Ser51, Sr53, Tyr171 and Gln212), two D XX ED motifs in domains II and IV, and the NADPH-binding residues were determined to be key for catalytic activity (see Supplementary Fig. 18 ) [29] . All of these catalytic residues and motifs are also conserved in both the LSS and LOS enzymes ( Supplementary Fig. 18 ), making it difficult at this time to determine which domains/residues are specific for LOS activity in a comparison of LSS and LOS. For initial characterization of the enzymatic activity of LSS and LOS, both proteins were expressed in Escherichia coli and the purified recombinant proteins tested for enzyme activity. LSS was shown to yield squalene as its sole product in an in vitro assay with FPP as the substrate, as expected ( Fig. 3a,b (I)). However, purified recombinant LOS incubated with GGPP in an in vitro assay showed lycopaoctaene as the sole reaction product ( Fig. 3a,b (II)). As LOS may have arisen from an SS paralogue that evolved to accept GGPP as substrate for lycopaoctaene production, we considered that LOS may have retained the ability to use FPP to produce squalene. Indeed, squalene production was detected when LOS was incubated with FPP in an in vitro reaction ( Fig. 3a,b (III)). More surprising, LOS incubation with PPP yielded lycopadiene, albeit at levels much lower than lycopaoctaene or squalene ( Fig. 3a,b (IV)). Similar in vitro incubations of LSS with GGPP or PPP did not result in lycopaoctaene or lycopadiene production (see below). As LOS can use three different substrates, steady-state kinetic experiments were performed with FPP, GGPP and PPP, to analyse LOS substrate specificity. The LOS enzyme shows higher substrate affinity ( K m ) for GGPP compared with that of FPP and PPP, and the turnover number ( k cat ) and catalytic efficiency ( k cat / K m ) for PPP are an order of magnitude less than for FPP and GGPP ( Table 1 and Supplementary Fig. 19 ). 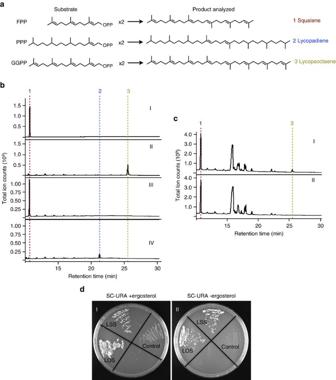Figure 3: Functional characterization of SSL enzymes from race Lin vitroandin vivo. (a) Diagram of reactions showing substrates and products for the analysis inbandc. (b) GC–MS profiles of LSS and LOSin vitroreaction products: I, LSS products using FPP as substrate to produce squalene (1); II, LOS products using GGPP as substrate to produce lycopaoctaene (3); III, LOS products using FPP as substrate to produce squalene (1); and IV, LOS products using PPP as substrate to produce lycopadiene (2). (c) GC–MS profiles of LOS yeastin vivoreaction products: I,n-hexane extractable metabolites of yeast expressingAtGGPPS11 and LOS, to make lycopaoctaene (3); or II, yeast expressingAtGGPPS11 alone. (d) Expression of LSS and LOS in theSS(ERG9) yeast knockout strain: I, in the presence of ergosterol, or II, in the absence of ergosterol, to test restoration of ergosterol prototrophy. The control carries the expression vector without a transgene. Data shown inb,canddare representatives from three independent experiments (n=3). Figure 3: Functional characterization of SSL enzymes from race L in vitro and in vivo . ( a ) Diagram of reactions showing substrates and products for the analysis in b and c . ( b ) GC–MS profiles of LSS and LOS in vitro reaction products: I, LSS products using FPP as substrate to produce squalene (1); II, LOS products using GGPP as substrate to produce lycopaoctaene (3); III, LOS products using FPP as substrate to produce squalene (1); and IV, LOS products using PPP as substrate to produce lycopadiene (2). ( c ) GC–MS profiles of LOS yeast in vivo reaction products: I, n -hexane extractable metabolites of yeast expressing At GGPPS11 and LOS, to make lycopaoctaene (3); or II, yeast expressing At GGPPS11 alone. ( d ) Expression of LSS and LOS in the SS ( ERG9 ) yeast knockout strain: I, in the presence of ergosterol, or II, in the absence of ergosterol, to test restoration of ergosterol prototrophy. The control carries the expression vector without a transgene. Data shown in b , c and d are representatives from three independent experiments ( n =3). Full size image Table 1 LOS steady-state kinetic parameters for GGPP, FPP and PPP substrates. Full size table To further characterize LOS, it was coexpressed in yeast with Arabidopsis thaliana GGPP synthase-11 ( At GGPPS11) [30] , as unlike FPP, yeast GGPP biosynthesis is limited and is considered a bottleneck for GGPP-derived isoprenoid production [31] . Coexpression of LOS and At GGPPS11 in yeast resulted in lycopaoctaene production ( Fig. 3c (I)), which was undetectable when At GGPPS11 was expressed without LOS ( Fig. 3c (II)). Furthermore, when expressed in a yeast SS knockout strain, LOS restored ergosterol prototrophy, indicating its ability to produce squalene in vivo ( Fig. 3d (I,II)). LSS was also able to restore ergosterol prototrophy as expected ( Fig. 3d (I,II)). Taken together, the results in Fig. 3 suggest LSS is a true SS enzyme, whereas LOS appears to be a promiscuous SSL enzyme with broader substrate chain length and saturation specificity. Previous studies have reported the production of lycopaoctaene (a.k.a. lycopersene) in vitro from protein extracts during studies conducted to decipher the carotenoid biosynthetic pathway [32] , [33] , [34] ; however, subsequent studies determined lycopaoctaene could not be an intermediate in carotenoid biosynthesis [35] , [36] , raising the possibility that lycopaoctaene production in these studies was an in vitro artefact. A more relevant study reported the ability of purified yeast SS to use GGPP for lycopaoctaene production in vitro , at levels much lower than native squalene production [32] . Importantly, we did not detect any lycopaoctaene production when At GGPPS11 was expressed alone in wild-type yeast ( Fig. 3c (II)), suggesting that yeast SS does not use GGPP in vivo under the conditions employed. Similarly, the ability of LOS to catalyse the conversion of PPP to lycopadiene may not have biological significance as we did not detect lycopadiene production using PPP as the substrate ex vivo in race L cell lysates ( Fig. 2b ) and the efficiency of LOS to use PPP as a substrate is quite low ( Table 1 ). Together, these results suggest that the relevant in vivo route to lycopadiene production is unlikely to involve the condensation of two PPP molecules by LOS, but rather, as we contend, the condensation of two GGPP molecules to form lycopaoctaene, for eventual conversion to lycopadiene. LOS is promiscuous towards prenyl substrates The LOS enzyme was further characterized using combinations of FPP, GGPP and PPP as substrates in in vitro reactions. Interestingly, in the presence of FPP and GGPP, LOS produced significant amounts of squalene and a C 35 H 58 molecule, and lesser amounts of lycopaoctaene ( Fig. 4a (I)). The C 35 H 58 molecule is a chimera produced from head-to-head condensation of one FPP molecule and one GGPP molecule, and its identity was confirmed by GC–MS ( Supplementary Fig. 20 ). Next, when LOS was supplied with FPP and PPP, squalene production predominated with small amounts of C 35 H 64 and lycopadiene ( Fig. 4a (II)). C 35 H 64 , also a chimeric hydrocarbon, is produced as a result of head-to-head condensation of one molecule each of FPP and PPP. Finally, LOS incubation with GGPP and PPP produced lycopadiene and lycopapentaene as minor products and lycopaoctaene as the major product ( Fig. 4a (III)). 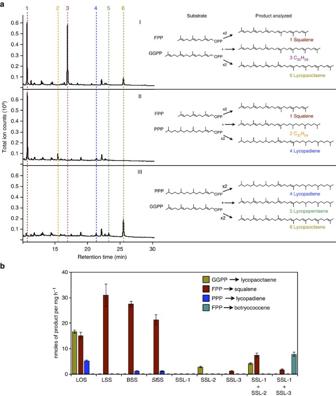Figure 4: Characterization of substrate use for SS and SSL enzymes. (a) Diagram of reactions showing substrates and products, and GC–MS profiles of LOS enzyme assay products with: I, FPP and GGPP substrates to produce squalene (1), C35H58(3) and lycopaoctaene (6); II, FPP and PPP substrates to make squalene (1), C35H64(2) and lycopadiene (4); and III, GGPP and PPP substrates to produce lycopadiene (4), lycopapentaene (5) and lycopaoctaene (6). Data shown are representatives from three independent experiments (n=3). (b) Radioactive enzyme assays using3H substrates GGPP, FPP and PPP with selected SS or SSL enzymes. SSL-1 produces PSPP from FPP substrate; however, PSPP was not analysed for in this assay. BSS, race B SS; LOS, lycopaoctaene synthase; LSS, race L SS;SlSS, SS fromS. lycopersicum(tomato), and SSL-1, SSL-2, SSL-3 are SSL enzymes from the B race ofB. braunii. Values shown are the mean±s.e. obtained from three independent measurements (n=3). Figure 4: Characterization of substrate use for SS and SSL enzymes. ( a ) Diagram of reactions showing substrates and products, and GC–MS profiles of LOS enzyme assay products with: I, FPP and GGPP substrates to produce squalene (1), C 35 H 58 (3) and lycopaoctaene (6); II, FPP and PPP substrates to make squalene (1), C 35 H 64 (2) and lycopadiene (4); and III, GGPP and PPP substrates to produce lycopadiene (4), lycopapentaene (5) and lycopaoctaene (6). Data shown are representatives from three independent experiments ( n =3). ( b ) Radioactive enzyme assays using 3 H substrates GGPP, FPP and PPP with selected SS or SSL enzymes. SSL-1 produces PSPP from FPP substrate; however, PSPP was not analysed for in this assay. BSS, race B SS; LOS, lycopaoctaene synthase; LSS, race L SS; Sl SS, SS from S. lycopersicum (tomato), and SSL-1, SSL-2, SSL-3 are SSL enzymes from the B race of B. braunii . Values shown are the mean±s.e. obtained from three independent measurements ( n =3). Full size image To the best of our knowledge, this is the first report where a wild-type, non-mutated eukaryotic SS or SSL enzyme has been shown to be able to use three naturally occurring prenyl diphosphate substrates to yield hydrocarbon products in all possible combinations. To support this notion, several SS and SSL enzymes were tested for their ability to use FPP, GGPP and PPP as substrates ( Fig. 4b ). The enzymes tested included LOS and three typical SS enzymes: LSS, BSS and Sl SS. In addition, enzymes SSL-1, SSL-2 and SSL-3 from race B were chosen because of their SSL activities. SSL-1 uses FPP to produce PSPP, which is then converted by SSL-2 to squalene, or by SSL-3 to C 30 -botryococcene as the major product and squalene as a minor product [37] . As shown in Fig. 4b , the typical SS enzymes display SS activity as their main catalytic function, with BSS and Sl SS also using PPP to produce minute amounts of lycopadiene. In contrast, the B race SSL enzymes have limited substrate flexibility, allowing SSL-2 and SSL-1 plus SSL-2 to use GGPP to generate minor amounts of lycopaoctaene ( Fig. 4b ). However, LOS is the only enzyme tested that is able to use all three substrates and to produce significant amounts of lycopaoctaene, squalene and lycopadiene ( Fig. 4b ). The LOS reaction uses a cyclopropyl intermediate We next conducted enzyme assays to determine whether the LOS reaction mechanism with GGPP as substrate is similar to that of SS, that is, uses a PSPP-like cyclopropyl diphosphate intermediate, which is termed prelycopaoctaene diphosphate (PLPP; Fig. 5a ). First, assays were conducted with or without a dinucleotide reducing agent, which would be required to convert PLPP to lycopaoctaene ( Fig. 5a ). LOS successfully used both NADH and NADPH as reducing agents for lycopaoctaene production, with preference for NADPH ( Fig. 5b ). In the absence of a dinucleotide reducing agent, LOS activity was lost ( Fig. 5b ), suggesting the presence of the PLPP reaction intermediate. This result is consistent with previous reports where yeast SS used GGPP in vitro to produce lycopaoctaene; however, without NADH or NADPH only the reaction intermediate PLPP accumulated [32] . Next, we showed that LOS is strongly inhibited by squalestatin ( Fig. 5c ), a potent SS inhibitor that mimics PSPP binding [23] , [38] , [39] , [40] . Finally, we identified PLPP as a reaction intermediate by conducting a GGPP-based LOS assay in the absence of NADPH, followed by acid phosphatase treatment to convert PLPP to prelycopaoctaene alcohol (PLOH). Analysis by GC–MS showed the presence of PLOH ( Fig. 5d ) with a fragmentation pattern consistent with previous reports of PLOH ( Supplementary Fig. 21 ) [32] . Taken together, these results are consistent with a two-step LOS reaction to produce lycopaoctaene. By analogy to SS, LOS catalyses the condensation of two GGPP units in the first half reaction to form the cyclopropylcarbinyl diphosphate intermediate PLPP, with concomitant release of one molecule of inorganic pyrophosphate ( Fig. 5a ). In the second half reaction, the PLPP cyclopropyl ring is cleaved and rearranged to form a 1-1′ linkage and further reduction by NADPH forms lycopaoctaene ( Fig. 5a ). 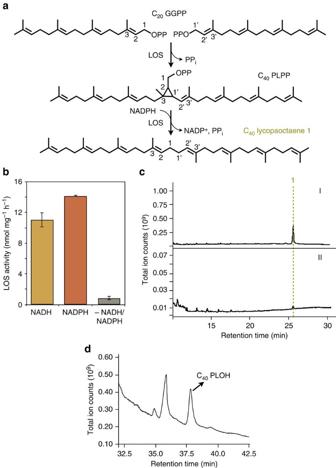Figure 5: Characterization of the LOS reaction intermediate. (a) Proposed LOS reaction mechanism to produce the PLPP intermediate and lycopaoctaene final product. (b) Radioactive LOS enzyme assays conducted with3H-GGPP substrate with or without NADH or NADPH reducing agents. Values shown are the mean±s.e. obtained from three independent measurements (n=3). (c) GC–MS profiles of LOS enzyme assay with GGPP as substrate to produce lycopaoctaene (1): I, in the absence, or II, in the presence of 20 nM squalestatin. (d) GC–MS profile of products from LOS enzyme assay with GGPP substrate in the absence of NADPH to produce PLPP, which was hydrolysed by acid phosphatase to yield PLOH for GC–MS analysis. Data shown incanddare representatives from three different experiments (n=3). Figure 5: Characterization of the LOS reaction intermediate. ( a ) Proposed LOS reaction mechanism to produce the PLPP intermediate and lycopaoctaene final product. ( b ) Radioactive LOS enzyme assays conducted with 3 H-GGPP substrate with or without NADH or NADPH reducing agents. Values shown are the mean±s.e. obtained from three independent measurements ( n =3). ( c ) GC–MS profiles of LOS enzyme assay with GGPP as substrate to produce lycopaoctaene (1): I, in the absence, or II, in the presence of 20 nM squalestatin. ( d ) GC–MS profile of products from LOS enzyme assay with GGPP substrate in the absence of NADPH to produce PLPP, which was hydrolysed by acid phosphatase to yield PLOH for GC–MS analysis. Data shown in c and d are representatives from three different experiments ( n =3). Full size image Our studies identified the first committed step in lycopadiene biosynthesis in race L of B. braunii and describe a new SSL enzyme, LOS, which carries out this reaction. Importantly, this enzyme may be used to engineer the effective production of hydrocarbon biofuel feedstocks in other photosynthetic or heterotrophic organisms in the future. This novel enzyme produces the tetraterpenoid lycopaoctaene from GGPP in a reaction analogous to that of SS. Lycopaoctaene would then undergo sequential reduction by a yet-to-be identified reductase enzyme(s) to form lycopahexaene, lycopapentaene, lycopatetraene, lycopatriene and finally lycopadiene as the major hydrocarbon product of the pathway ( Fig. 6 ). Furthermore, we show that the wild-type LOS enzyme displays remarkable substrate flexibility and can use at least three different, naturally occurring C 15 and C 20 prenyl diphosphate substrates in vivo and in vitro for the combinatorial biosynthesis of hydrocarbons belonging to three terpene classes: triterpenes, sesquarterpenes and tetraterpenes. 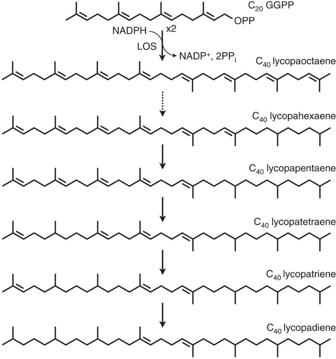Figure 6: Proposed pathway for lycopadiene biosynthesis. LOS uses GGPP in a two-step reaction to produce lycopaoctaene, which is further reduced by a yet unknown enzyme(s) to produce lycopahexaene, lycopapentaene, lycopatetraene, lycopatriene and finally lycopadiene. Figure 6: Proposed pathway for lycopadiene biosynthesis. LOS uses GGPP in a two-step reaction to produce lycopaoctaene, which is further reduced by a yet unknown enzyme(s) to produce lycopahexaene, lycopapentaene, lycopatetraene, lycopatriene and finally lycopadiene. Full size image When used under artificial reaction conditions, other SSL enzymes have been described to show relaxed substrate flexibility and to yield products of varying lengths. One such enzyme is CrtM, a dehydrosqualene synthase from Staphylococcus aureus that is involved in C 30 carotenoid biosynthesis [41] , [42] , [43] . In S. aureus and also when overexpressed in E. coli , CrtM uses two FPP molecules to produce dehydrosqualene, a C 30 squalene-like molecule with a cis double bond at the 1-1′ linkage of the two FPP molecules [44] . Expression of a GGPP synthase in E. coli also expressing CrtM led to the depletion of FPP and the overproduction of GGPP [41] . Under these conditions, CrtM was found to generate its native C 30 product, a C 35 homologue and C 40 phytoene, indicating the ability of CrtM to accept GGPP as a substrate when the natural FPP substrate is limiting [41] . CrtM was further engineered through mutations to accept C 25 farnesylgeranyl diphosphate, yielding C 40 , C 45 and C 50 homologues of dehydrosqualene in the presence of FPP, farnesylgeranyl diphosphate and GGPP [42] , [43] . In another study, SSs from yeast, pig and rat have been shown to accept non-natural derivatives of FPP, to generate several unnatural terpene products in vitro [45] , [46] . In addition, yeast SS has been shown to yield alternative products in vitro from FPP as a substrate under various non-physiological reaction conditions, such as in the absence of NADPH with extended incubation times or in the presence of an unreactive NADPH analogue [47] , [48] , [49] . Irrespective of these examples, the promiscuity of LOS is still remarkable, considering that the wild-type LOS enzyme is able to accept three naturally occurring prenyl diphosphate substrates and produce the chimeric hydrocarbons described here without the need for mutations or altered, non-physiological reaction conditions. Such remarkable intrinsic substrate promiscuity has not been documented for any other eukaryotic SS or SSL enzyme up until now. Ours and other studies [37] , [50] raise the question about how SSL enzymes arise. LSS and LOS from B. braunii share >50% sequence identity and both contain the important catalytic residues and conserved domains of SS enzymes ( Supplementary Fig. 18 ), but they still have different substrate preferences and product formation. Thus, we hypothesize that an ancient SS gene may have undergone gene duplication in race L. The paralogue that gave rise to LSS maintained the ability to produce squalene as its sole product to support sterol biosynthesis for primary metabolism. However, the paralogue that yielded LOS developed the use of alternative substrates for hydrocarbon oil production, while also preserving SS activity. A similar scenario has been suggested as a possible mechanism for generating new secondary metabolites that may provide a fitness benefit to the host organism [42] , [51] . For B. braunii , it has been proposed that hydrocarbon oils and their derivatives increase the buoyancy of colonies for increased exposure to sunlight [50] , [52] , [53] . Similar gene diversifications have also been proposed in the B race of B. braunii for botryococcene production, and in some bacteria for squalene generation. For botryococcene production, SS duplications gave rise to the SSL-1 and SSL-3 genes/enzymes responsible for botryococcene production, while retaining a residual ability to produce squalene [37] . For bacteria, a three-enzyme system for squalene production arose from successive gene duplication events [50] . LOS produces a variety of terpenes in vitro when offered a mixture of substrates and may likely also do so in vivo . In the in vitro mixed substrate assays with LOS ( Fig. 4a ), a C 35 H 64 molecule was observed from FPP and PPP condensation. This product has the exact same GC retention time and mass spectrum as the C 35 H 64 hydrocarbon detected in the total hydrocarbon pool ( Fig. 2a (VII) and Fig. 4a (II)). This suggests that LOS is also promiscuous in B. braunii cells, but at best has limited access to the FPP and PPP pools, as the C 35 H 64 product only comprises 0.15% of the total hydrocarbons ( Fig. 2a (VII)). The FPP–GGPP condensation product C 35 H 58 seen in these in vitro assays ( Fig. 4a (I)) is not detected in the total hydrocarbon pool, possibly because this molecule is reduced to C 35 H 64 in vivo . It should be noted that two previous studies described several C 35 squalene-like isoprenoids from Methanococcus jannaschii and Thermococcus barophilus , including the C 35 H 58 and C 35 H 64 molecules identified here [54] , [55] , although the enzymatic basis for the biosynthesis of these products remains uncharacterized. In addition, the ability of LOS to produce lycopapentaene as an observed in vitro condensation product of GGPP and PPP ( Fig. 4a (III)) may indicate the existence of an alternative in vivo biosynthetic route to this molecule and may be partially responsible for the relative prevalence of lycopapentaene (3% of total hydrocarbons; Fig. 2a (IV)) among the minor hydrocarbons of race L. This would suggest that LOS can also use PPP in vivo . However, LOS does not appear to use PPP as a single substrate for lycopadiene production in vivo , as we were not able to detect lycopadiene synthesis activity in cell fractions using PPP as substrate ( Fig. 2b ). The promiscuous LOS described in this work is nevertheless used by B. braunii Race L to produce lycopaoctaene preferentially over squalene, as shown by the large amounts of hydrocarbon oils produced by this alga and the absence of detectable amounts of squalene or non-sterol squalene derivatives in the total hydrocarbon pool. In contrast, accumulation of the non-sterol squalene derivatives methylsqualenes in race B are thought to arise from squalene produced by the additional enzyme SSL-2 (ref. 37 ). Thus, detection of non-sterol squalene derivatives in race L would be expected if LOS was producing squalene in vivo . We hypothesize that the observed preference of LOS for C 40 lycopaoctaene biosynthesis over C 30 squalene production in vivo may result from an increased flux from GGPP over FPP due to metabolic channelling, to form a biosynthetic metabolon specific for lycopadiene production. Formation of such metabolons is common in plants and is used for channelling substrates and intermediates required for the biosynthesis of different classes of plant natural products, including isoprenoids [56] , [57] , [58] . When expressed in yeast, LOS may produce squalene presumably due to a lack of this proposed metabolon, thus giving LOS access to the FPP pool. We therefore conclude that LOS is responsible for synthesizing lycopaoctaene as the first committed step towards lycopadiene hydrocarbon biosynthesis in race L of B. braunii . Reagents [1- 3 H]-FPP (specific activity, 18.2 Ci mmol −1 ) was purchased from PerkinElmer. [1- 3 H]-GGPP (specific activity, 20.0 Ci mmol −1 ), [1- 3 H]-PPP (specific activity, 20.0 Ci mmol −1 ) and non-radiolabelled PPP were purchased from American Radiolabeled Chemicals. When required, specific activities of radiolabelled chemicals were adjusted with non-labelled chemicals. Solvents and chemicals were purchased from VWR. All other reagents were purchased from Sigma unless otherwise noted. Culturing of B. braunii B. braunii , race L, Songkla Nakarin strain [16] was obtained from Algobank-Caen Microalgal Culture Collection, University of Caen Basse-Normandie, France, and grown in a modified Chu 13 medium, pH 7.5 (ref. 59 ) at 22 °C under continuous aeration of filter-sterilized air enriched with 2.5% CO 2 . The concentrations of chemicals in modified Chu 13 medium were as follows: KNO 3 (0.4 g l −1 ), MgSO 4 ·7H 2 O (0.1 g l −1 ), K 2 HPO 4 (0.052 g l −1 ), CaCl 2 ·2H 2 O (0.054 g l −1 ), FeNa EDTA (0.01 g l −1 ), H 3 BO 4 (2.86 mg l −1 ), MnSO 4 ·H 2 O (1.54 mg l −1 ), ZnSO 4 ·7H 2 O (0.22 mg l −1 ), CuSO 4 ·5H 2 O (0.08 mg l −1 ), NaMoO 4 ·2H 2 O (0.06 mg l −1 ) and CoSO 4 ·7H 2 O (0.09 mg l −1 ). The cultures were grown under a 12:12 h light:dark cycle with a light intensity of 120 μE m −2 s −1 . Algae cells were subcultured by inoculation of 100 ml of a floating 6-week-old culture to 750 ml of fresh medium. Hydrocarbon staining and microscopy Nile Red (Sigma) staining of L race hydrocarbons was done by treating 500 μl of B. braunii L race colonies in medium at early phase (5 day) density with 2.5 μl of a stock solution of Nile Red dissolved in acetone (0.15 mg ml −1 ) for a final concentration of Nile red of 0.375 g ml −1 and acetone of 0.25%. Samples were kept in the dark and incubated at room temperature for 15 min before imaging. Confocal microscopy images were obtained using an Olympus IX83-FV1200 inverted confocal microscope with spectral detection unit using an Olympus UPLSAPO × 60 oil-immersion objective (numerical aperture=1.35). The confocal aperture diameter was set to 1 Airy disk unit and Z -series images were acquired with voxel dimensions of 101 × 101 × 490 (nm; x - y - z , respectively). Nile Red and chlorophyll were excited using a 488-nm laser and detected using 540–590 nm and 655–755 nm barrier filter settings, respectively. Bright-field images were acquired via the transmitted detector using the 488-nm laser. Maximum intensity projections and brightness/contrast adjustments were completed using the Olympus FV-ASW software version 4. Hydrocarbon purification Hydrocarbons were purified as described previously [60] , [61] and as follows. Algal cells were harvested by vacuum filtration using a 10-μm nylon-mesh filter, freeze-dried, extracted twice with n -hexane for 2 h, to recover extracellular hydrocarbons, and then twice with CHCl 3 :MeOH (2:1) for 12 h stirring at room temperature, to recover intracellular hydrocarbons. Both extracts were concentrated separately using a rotary evaporator and resuspended in a small amount of n -hexane before running through separate gravity-fed silica gel columns with n -hexane as solvent. The n -hexane eluent before the pigment front was collected as the hydrocarbon fraction. Both extracellular and intracellular hydrocarbon fractions were combined and evaporated to dryness, to recover the total hydrocarbon pool of the algae. Individual hydrocarbon molecules were purified by injecting the total hydrocarbon sample onto an HPLC Develosil 60 silica column (20 mm × 250 mm) using n -hexane as a mobile phase at a flow rate of 6 ml min −1 and detection at 210 nm. An aliquot of the purified hydrocarbons were analysed by GC–MS for purity analysis. GC–MS conditions Enzyme assay products, purified hydrocarbons and yeast extracts were analysed by GC–MS (Bruker 436-GC-SCION SQ Premium) using a 5% Phenyl BR-5 ms capillary column (30 m × 0.25 mm, film thickness: 0.25 μm) in electron ionization (70 eV) mode. Initial oven temperature was 220 °C, held for 1 min, then increased to 280 °C at the rate of 5 °C min −1 and then ramped to 300 °C at a rate of 2 °C min −1 and held for 20 min. Helium was used as a carrier gas at a flow rate of 2.58 ml min −1 . Temperatures of injection port, interface and ion source were 280 °C, 250 °C and 200 °C, respectively. Hydrocarbon NMR analysis One-dimensional NMR spectra of race L hydrocarbons molecules suffer from severe spectral overlap and the data interpretation is further complicated by degenerate chemical shifts as a result of symmetry planes in the lycopadiene structure. Consequently, hetero-nuclear two-dimensional (2D) experiments were used for unambiguous structural characterization of each entity. NMR experiments were performed at 25 °C on purified samples dissolved in deuterated chloroform using a 500 MHz Bruker Avance III HD spectrometer equipped with an inverse detection TXI probe. We have relied on 2D heteronuclear experiments acquired at natural abundance of 13 C nuclei, to deduce structures of these molecules. Multiplicity-edited 2D heteronuclear single quantum coherence spectrum was acquired for each compound and the resonances were assigned using a combination of 2D heteronuclear 2 bond correlation, 2D heteronuclear multiple bond correlation and 2D heteronuclear single quantum coherence–total correaltion spectroscopy experiments. The 13 C chemical shifts obtained for lycopadiene match those previously obtained [16] . Spectral data for hydrocarbons analysed Lycopadiene: 1 H NMR (500 MHz, CDCl 3 ): δ 0.87, 0.89, 1.08, 1.09, 1.16, 1.2, 1.29, 1.39, 1.4, 1.54, 1.61, 1.96, 2.04, 2.17, 5.15; 13 C NMR (125 MHz, CDCl 3 ): δ 15.9, 19.7, 22.7, 24.5, 24.7, 25.4, 28.0, 28.3, 31.2, 32.8, 36.8, 37.4, 39.4, 40.0, 124.0, 135.9; MS ( m/z ): [M + ] calcd. for C 40 H 78 , 558.61; found, 558.70. Lycopatriene: 1 H NMR (500 MHz, CDCl 3 ): δ 0.87, 0.89, 1.08, 1.09, 1.13, 1.16, 1.2, 1.29, 1.29, 1.39, 1.4, 1.54, 1.61, 1.63, 1.71, 1.96, 1.98, 2.04, 2.16, 5.12, 5.15; 13 C NMR (125 MHz, CDCl 3 ): δ 15.9, 17.6, 19.7, 22.7, 24.5, 24.7, 24.7, 25.4, 25.6, 25.7, 28.0, 28.3, 30.8, 32.7, 36.8, 37.1, 37.4, 39.4, 40.0, 124.1, 125.1, 131.1, 135.9; MS ( m/z ): [M + ] calcd. for C 40 H 76 , 556.59; found, 556.70. Lycopatetraene: 1 H NMR (500 MHz, CDCl 3 ): δ 0.87, 0.89, 1.08, 1.13, 1.16, 1.2, 1.29, 1.39, 1.4, 1.54, 1.61, 1.63, 1.71, 1.95, 1.96, 1.99, 2.04, 2.16, 5.12, 5.15; 13 C NMR (125 MHz, CDCl 3 ): δ 15.9, 17.6, 19.7, 22.7, 24.5, 24.7, 25.4, 25.5, 25.7, 28.0, 28.3, 30.8, 32.7, 36.6, 37.1, 37.4, 39.3, 39.4, 40.0, 124.1, 125.2, 131.1, 135.9; MS ( m/z ): [M + ] calcd. for C 40 H 74 , 554.58; found, 554.60. Lycopapentaene: 1 H NMR (500 MHz, CDCl 3 ): δ 0.87, 0.89, 1.08, 1.16, 1.2, 1.29, 1.39, 1.4, 1.55, 1.62, 1.63, 1.71, 2, 2.04, 2.09, 2.23, 5.15; 13 C NMR (125 MHz, CDCl 3 ): δ 16.0, 17.7, 19.8, 22.7, 24.5, 24.7, 25.4, 25.7, 26.7, 28.0, 28.3, 31.0, 32.8, 36.6, 37.4, 39.4, 39.8, 124.2, 131.1, 135.9; MS ( m/z ): [M + ] calcd. for C 40 H 72 , 552.56; found, 552.70. Lycopapentaene isomer: 1 H NMR (500 MHz, CDCl 3 ): δ 0.87, 0.89, 1.08, 1.13, 1.16, 1.2, 1.29, 1.4, 1.55, 1.62, 1.63, 1.71, 1.99, 2, 2.04, 2.09, 5.1, 5.15; 13 C NMR (125 MHz, CDCl 3 ): δ 16.0, 17.7, 19.8, 22.7, 24.5, 24.7, 25.5, 25.7, 26.7, 28.0, 28.3, 32.7, 36.6, 37.1, 37.4, 39.4, 39.8, 124.2, 124.8, 131.1, 135.9; MS ( m/z ): [M + ] calcd. for C 40 H 72 , 552.56; found, 552.90. Lycopahexaene: 1 H NMR (500 MHz, CDCl 3 ): δ 0.87, 0.89, 1.08, 1.16, 1.2, 1.29, 1.4, 1.55, 1.61, 1.63, 1.71, 1.96, 1.99, 2.04, 2.06, 5.15; 13 C NMR (125 MHz, CDCl 3 ): δ 16.0, 17.7, 19.8, 22.7, 24.5, 24.7, 25.7, 26.8, 28.0, 28.3, 32.8, 36.6, 37.4, 39.4, 39.8, 124.3, 131.1, 135.9; MS ( m/z ): [M + ] calcd. for C 40 H 70 , 550.55; found, 550.60. Lycopaoctaene: 1 H NMR (500 MHz, CDCl 3 ): δ 1.62, 1.63, 1.71, 2, 2.03, 2.04, 5.15; 13 C NMR (125 MHz, CDCl 3 ): δ 16.0, 17.7, 25.7, 27.2, 28.3, 39.8, 124.3, 131.1, 135.9; MS ( m/z ): [M + ] calcd. for C 40 H 66 , 546.52; found, 546.70. C 35 H 64 : 1 H NMR (500 MHz, CDCl 3 ): δ 0.83, 0.86, 1.06, 1.13, 1.19, 1.21, 1.24, 1.32, 1.36, 1.52, 1.61, 1.68, 1.98, 2.01, 2.06, 5.13; 13 C NMR (125 MHz, CDCl 3 ): δ 16.3, 17.9, 20.0, 22.9, 24.4, 24.8, 25.1, 26.0, 26.3, 27.2, 28.2, 33.0, 37.7, 39.6, 40.0, 124.8, 131.4, 135.1; MS ( m/z ): [M + ] calcd. for C 35 H 64 , 484.50; found, 484.70. Ozonolysis experiments Owing to the limited amount of minor hydrocarbons in the total L race hydrocarbon pool, ozonolysis experiments were conducted only on those hydrocarbons that could be purified to obtain at least 10 mg: lycopadiene, lycopatriene and lycopapentaene. These hydrocarbons were separately dissolved in dichloromethane and submitted to ozone cleavage for 5 min at −78 °C. Each product from reductive cleavage of the resulting ozonide was directly subjected to GC–MS (electron ionization) analyses without purification. GC–MS analysis was carried out using a GCMS-QP2010 Ultra spectrometer (Shimadzu, Kyoto, Japan) equipped with a capillary column (InertCap 1MS, GL Science; 60 m × 0.25 mm, film thickness: 0.25 μm). The column temperature was programmed as follows: 50 °C for 1 min, raised at 10 °C min −1 from 50 to 220 °C, then at 2 °C min −1 from 220 to 260 °C and held for 22 min at the final temperature. Helium was used as a carrier gas at a flow rate of 41.2 cm s −1 . Temperatures of injection port, interface and ion source were 260, 250 and 200 °C, respectively. Preparation of algal cell lysate Algae from the rapid growth phase were harvested, snap frozen with liquid nitrogen and stored at −80 °C for future use. In a typical preparation, 200 mg of frozen algae was added to eight individual tubes containing 0.8 ml extraction buffer (50 mM MOPS pH 6.8, 20 mM MgCl 2 , 5 mM β-mercaptoethanol, 5 mM EGTA and 20% (v/v) glycerol) with 200 μl of stainless steel metal beads (mixture of 0.9–2 mm diameter beads) and then homogenized using a Bullet Blender Storm 24 (Next Advance, Inc., USA) for 10 min at a speed of 10. The algal homogenates were centrifuged at 9,000 g for 10 min at 4 °C. The 9,000 g supernatants were pooled and then centrifuged at 100,000 g for 1 h to obtain the soluble fraction. The pellet was washed with 4 ml extraction buffer and centrifuged again at 100,000 g . This process was repeated twice and the pellet was resuspended in 0.5 ml extraction buffer to obtain a microsomal fraction. An aliquot of each protein fraction was used for enzyme assays. Enzyme assays Radioactive enzyme assays were conducted in a 50-μl total reaction volume as described previously [23] , [37] and as follows. Reactions were initiated by adding 10 μg algal lysate or 1 μg of recombinant enzyme purified from E. coli to a reaction buffer containing 50 mM MOPS pH 6.8, 2.5 mM β-mercaptoethanol, 20 mM MgCl 2 , 2 mM NADPH or NADH and 10 μM [1- 3 H]-prenyl-PP substrate (specific activity=0.25 Ci mmol −1 ). Enzyme assays were incubated at 37 °C for 60 min and terminated by adding 60 μl of n -hexane, followed by brief vortexing and centrifugation. Thirty microlitres of the organic layer was spotted onto silica gel 60 thin-layer chromatography plates along with authentic standards of squalene ( R f =0.17), C 30 -botryococcene ( R f =0.2), lycopaoctaene ( R f =0.09) and lycopadiene ( R f =0.5), and then developed with n -hexane. Hydrocarbon standards were visualized by iodine vapour and spots corresponding to authentic standards were scraped and analysed by liquid scintillation counter, to determine radioactive incorporation into the respective hydrocarbons. SS and botryococcene synthase assays were conducted using 3 H-FPP, whereas LOS and lycopadiene synthase assays were conducted using 3 H-GGPP and 3 H-PPP, respectively. For GC–MS analysis of reaction products, enzyme assays were conducted with non-radiolabelled substrates in glass vials by scaling the total reaction volume and contents to 500 μl. Two separate 500 μl reactions were each extracted twice with 1 ml n -hexane, the extracts pooled, dried under a stream of nitrogen gas, resuspended in 100 μl n -hexane and a 5-μl aliquot analysed by GC–MS. Hydrocarbon accumulation and LOS activity over growth cycle Several flasks of race L culture were grown over a 39- day culture period. Twenty-five millilitres of culture was collected at indicated times on pre-weighed Whatman GF/C filters by vacuum filtration. The filters with algae were dried in an 80 °C oven and total hydrocarbons were extracted using the protocol described above. Similarly, 500 ml of algae cells were also harvested at indicated times by filtering through a 10-μm nylon mesh and the samples used to determine LOS enzyme activity over the culture period. LOS enzyme assays were conducted using 10 μg of 9,000 g supernatant. RNA isolation Total RNA was isolated as previously described [62] and as follows. For B. braunii , liquid nitrogen frozen samples were pulverized using a Tissuelyser II (Qiagen, Valencia, CA). Approximately 200 mg of this frozen pulverized B. braunii tissue, or frozen leaf tissues of A. thaliana and S. lycopersicum , were ground in a mortar and pestle with liquid nitrogen. The samples were then added to 1 ml of TRIzol (Life Technologies, Grand Island, NY) and the total RNA was isolated following the manufacturer’s instructions. The RNA from A. thaliana and S. lycopersicum were used directly for gene cloning (see below). For the B. braunii RNA, contaminating polysaccharides were removed before the use for gene cloning as follows. The RNA pellet was resuspended in 0.5 ml 2 M LiCl, incubated for 5 min and centrifuged at 12,000 g for 15 min at 4 °C to pellet the total RNA. The polysaccharides remain in the supernatant. This process was repeated until the size of RNA pellet remained constant. The RNA pellet was then dissolved in 0.5 ml 1 × Tris-EDTA (TE), extracted with an equal volume of phenol/chloroform/isoamyl alcohol mix (25:4:1) and centrifuged at 12,000 g for 15 min at 4 °C. The aqueous supernatant phase was removed and extracted with 0.5 ml of chloroform followed by centrifugation at 12,000 g for 15 min at 4 °C. The RNA was precipitated from the aqueous supernatant by adding 0.1 volume 3 M sodium acetate and 2.5 volumes of 100% ethanol, incubated for 20 min at −20 °C and centrifuged at 12,000 g for 15 min at 4 °C. The RNA pellet was washed twice with 0.5 ml 70% ethanol, centrifuged at 12,000 g for 15 min at 4 °C, the pellet dried using a speedvac and the RNA resuspended in 50 μl of RNAase-free water. LSS and LOS cloning RNAseq analysis on the L race of B. braunii was carried out as previously reported [62] and as follows. RNA isolated from days 0, 3, 7, 14, 21 and 28 over the 4-week culture cycle were kept separate, paired-end libraries were prepared from each RNA sample and each sample was sequenced under the Illumina platform. A transcriptome contig library was created using the Trinity software suite. SSL sequences were computationally screened using this transcriptomic database with BSS as a query. Two SSL cDNAs, LSS and LOS , were identified. Total RNA was extracted from a day-3 race L culture and first-strand cDNA was prepared using the SuperScript III first-strand synthesis kit (Invitrogen). Primers specific to each cDNA based on the transcriptome sequence were used to amplify the PCR product from first-strand cDNA using GoTaq DNA polymerase mix (Promega) followed by cloning into the pGEM-T vector (Promega). Gene-specific primers were as follows: For LSS , forward primer 5′- ATGGGGAAGCTACAGGAGGTTTTGAAGC -3′ and reverse primer 5′- TCAGGCAAGGCCGCCGCGAAG -3′; for LOS , forward primer 5′- ATGAAGTACACAGATTTCCTTGCGC -3′ and reverse primer 5′- TCACACAGTCTTGAGGGCGAG -3′. AtGGPPS11 and SlSS cloning The cDNA sequences for AtGGPPS11 ( At 4g36810) [30] and SlSS were obtained from the NCBI nucleotide database. Total RNA isolated from the leaves of A. thaliana and S. lycopersicum were used for first-strand cDNA synthesis and PCR products corresponding to each cDNA were amplified using gene-specific primers followed by cloning into the pGEM-T vector. Gene-specific primers used for PCR amplification were as follows: for AtGGPPS11 , forward primer 5′- ATGGCTTCAGTGACTCTAGGTTC -3′ and reverse primer 5′- TCAGTTCTGTCTATAGGCAATG -3′; for SlSS , forward primer 5′- ATGGGAACATTGAGGGCA -3′ and reverse primer 5′- CTAAGACCGGCTGCCAAAAAGTTG -3′. Protein expression and purification Except for SSL-1 and SSL-3 , DNA sequences encoding the predicted transmembrane domain at the carboxy terminus of each SS or SSL protein were deleted and then cloned to pET28a, to encode for amino terminal 6 × His-tagged proteins. DNA templates of BSS , SSL-1 , SSL-2 and SSL-3 were received from previous studies [25] , [37] . The pET28a expression constructs were made using appropriate restriction sites; LOS Δ391–444 with NheI and HindIII; LSS Δ399–462 , SlSS Δ387–411 , BSS Δ399–461 , SSL-1 and SSL-3 with NdeI and HindIII; and SSL-2 Δ392–465 with NdeI and SalI. The expression constructs were transformed into E. coli BL21(DE3), grown at 37 °C to OD 600 =0.8 and protein expression for each gene induced by adding 1 mM isopropylthio-β- D -galactoside. The induced cultures were then grown for an additional 6 h at 25 °C. His-tagged proteins were purified at 4 °C by standard procedures. In a typical purification, pellets from a 100-ml culture were resuspended in 10 ml extraction buffer (50 mM sodium phosphate buffer pH 7.8, 300 mM NaCl, 10 mM imidazole, 1 × general protease inhibitor cocktail (Sigma), 1 mM MgCl 2 and 1% glycerol (v/v)), and then sonicated four times for 15 s at 70% maximum power with 2 min interval between each sonication. The sonicated samples were centrifuged at 16,000 g for 10 min at 4 °C. The supernatants were applied to a gravity-fed column containing Ni-NTA agarose (Qiagen) and the His-tagged proteins were purified according to the manufacturer’s recommendations. The wash buffer (50 mM sodium phosphate buffer pH 7.8, 300 mM NaCl, 60 mM imidazole, 1 mM MgCl 2 and 1% glycerol (v/v)) and the elution buffer (50 mM sodium phosphate buffer pH 7.8, 300 mM NaCl, 400 mM imidazole, 1 mM MgCl 2 and 1% glycerol (v/v)) were used for protein purification. The eluted fractions were dialysed using storage buffer (300 mM NaCl, 20 mM Tris-HCl pH 7.5, 5 mM dithiothreitol and 2 mM MgCl 2 ), concentrated with an Amicon Ultra centrifugal filter (0.5 ml, 30 kDa cutoff; EMD Millipore) to desired protein concentration, an equal amount of 100% glycerol added and stored at −20 °C for 1–2 months without a loss of enzyme activity. LOS steady-state kinetic experiments Michaelis–Menten enzyme kinetics experiments with the LOS enzyme were set up using the protocol described previously [63] and as follows. Pilot experiments were initially conducted using radioactive enzyme assays, to determine the reaction conditions where reaction velocity is linear (<10% turnover) with respect to enzyme concentration. For steady-state kinetics experiments, enzyme assays (50 μl total reaction volume) were conducted with 100 nM of purified LOS enzyme at the indicated concentration of 3 H-GGPP, 3 H-FPP or 3 H-PPP for a set time interval. Kinetics for the NADPH cofactor were not determined and this factor was held constant at 2 mM in all assays. The reaction velocities were plotted against substrate concentrations to generate Michaelis–Menten curves and the kinetics parameters of LOS enzyme for GGPP, FPP and PPP were determined by analysing the data using GraphPad Prism 6 software. Yeast expression The DNA sequence encoding the 56 N-terminal amino acids for the plastid-targeting signal of AtGGPPS11 were deleted resulting in AtGGPPS11 Δ57 , which was cloned into pESC-TRP using BamHI and SalI restriction sites for expression under the inducible GAL1 promoter. For coexpression studies, the DNA sequences encoding the predicted C-terminal transmembrane domain of LOS was deleted resulting in LOS Δ391–444 , which was cloned into the second multiple cloning site of AtGGPPS11 Δ57 :pESC-TRP using EcoRI and SpeI restriction sites for expression under the inducible GAL10 promoter. The yeast expression constructs AtGGPPS11 Δ57 :pESC-TRP and AtGGPPS11 Δ57 + LOS Δ391–444 :pESC-TRP were introduced into yeast strain CKY457 ( MAT a , leu2Δ1, ura3-52 , trp1Δ63 , his3Δ200 and lys2-128 ) via lithium acetate transformation followed by selection on yeast synthetic dropout medium (SC-TRP). Positive transformants were grown at 30 °C in 150 ml SC-TRP media to mid-log phase, induced with 2% final galactose concentration and grown for an additional 130 h. Yeast cells were harvested, freeze-dried and extracted with n -hexane for 2 h by stirring at room temperature. The organic extracts were centrifuged at 1,000 g , the supernatant dried using a rotary evaporator, resuspended in 500 μl n -hexane and a 5-μl aliquot analysed by GC–MS to evaluate for the production of lycopaoctaene. Purification of lycopaoctaene standard A 3-l culture of yeast strain CKY457 expressing AtGGPPS11 Δ57 + LOS Δ391–444 :pESC-TRP was grown and the metabolites were extracted with n -hexane using the protocol described above. The organic extracts were applied to a silica gel gravity-fed column and metabolites eluted sequentially with two different solvent systems, n -hexane and 1% diethyl ether in n -hexane. The 1% diethyl ether in n -hexane eluent fraction containing lycopaoctaene and other metabolites was concentrated and resuspended in a small volume of n -hexane before injecting the samples onto a 10 mm × 250 mm Cosomil 5C 18 -AR-II HPLC column. Lycopaoctaene was purified by reversed phase HPLC using methanol:acetone (60:40) as a mobile phase at a flow rate of 3 ml min −1 and detection at 210 nm. Identity of lycopaoctaene molecule was confirmed by GC–MS ( Supplementary Fig. 3 ) and NMR ( Supplementary Table 1 and Supplementary Fig. 15 ). LSS and LOS complementation of yeast SS knockout strain The yeast strain ZX 178-08 ( MAT a , his3 , leu2 , met15 , ura3 , SUE and erg9Δ::HPH ), which has a knockout of the endogenous SS gene ( ERG9 ), was used for complementation experiments [64] . The expression vector XURA used in our study was made by replacing the GAL1 and GAL10 promoters in pESC-URA vector backbone with constitutive promoters TEF1 and GPD, respectively [65] . Full-length LSS was cloned into XURA using Not1 and SpeI restriction sites. Full-length LOS was cloned into EcoRI and SpeI sites of XURA vector. The expression constructs LSS :XURA, LOS :XURA and XURA were transformed into ZX 178-08 yeast strain via lithium acetate transformation followed by selection on yeast synthetic dropout medium supplemented with ergosterol synthetic complete-Uracil (SCE URA). The positive transformants were further characterized by streaking on selection media with or without ergosterol, to test the ability of individual genes to restore ergosterol prototrophy of ZX 178-08 yeast. GC–MS analysis of PLOH The enzyme assay for PLPP was conducted following the protocol described previously for analysis of PSPP [37] , [50] and as follows. The PLPP assay contained 50 mM MOPS (pH 6.8), 2.5 mM β-mercaptoethanol, 20 mM MgCl 2 , 180 μM GGPP and 750 μg of purified LOS enzyme in a 2.5-ml total reaction volume. The reaction mixture was incubated at 37 °C for 2 h and terminated by snap freezing with liquid nitrogen followed by lyophilization. For hydrolysis of PLPP to PLOH, the white residue obtained after lyophilization was resuspended in 2 ml phosphatase solution (20% 1-propanol, 100 mM sodium acetate pH 4.7, 0.1% Triton-X-100 and 50 units of sweet potato acid phosphatase) and then incubated for 16 h in a 28 °C shaker. The dephosphorylation reaction mixture was extracted three times with 4 ml of methyl tertiary butyl ether (MTBE), the extracts pooled, dried under a stream of nitrogen gas, resuspended in 100 μl n -hexane and a 5-μl aliquot analysed by GC–MS as under the conditions described above with the following differences. Chemical ionization using methane gas at 20 psi was employed for analysis of the PLOH molecule, as electronic ionization did not result in a molecular ion of PLOH. Initial oven temperature was 70 °C, held for 1 min, then increased to 200 °C at the rate of 8 °C min −1 and then ramped to 300 °C at a rate of 20 °C min −1 and held for 20.75 min. Temperatures of injection port, interface and ion source were 260 °C, 250 °C and 200 °C, respectively. Accessions codes : New DNA sequences described in this study have been deposited in GenBank: accession # KT388100 , accession # KT388101 and accession # NM_001247787 . How to cite this article: Thapa, H. R. et al . A squalene synthase-like enzyme initiates production of tetraterpenoid hydrocarbons in Botryococcus braunii Race L. Nat. Commun. 7:11198 doi: 10.1038/ncomms11198 (2016).